Excitonic quasiparticles in a spin–orbit Mott insulator In condensed matter systems, out of a large number of interacting degrees of freedom emerge weakly coupled quasiparticles (QPs), in terms of which most physical properties are described. The lack of identification of such QPs is a major barrier for understanding myriad exotic properties of correlated electrons, such as unconventional superconductivity and non-Fermi liquid behaviours. Here we report the observation of a composite particle in a quasi-two-dimensional spin–1/2 antiferromagnet Sr 2 IrO 4 —an exciton dressed with magnons—that propagates with the canonical characteristics of a QP: a finite QP residue and a lifetime longer than the hopping time scale. The dynamics of this charge-neutral excitation mirrors the fundamental process of the analogous one-hole propagation in the background of spins–1/2, and reveals the same intrinsic dynamics that is obscured for a single, charged-hole doped into two-dimensional cuprates. The dynamics of a single hole doped into a low-dimensional quantum antiferromagnet (AF) constitutes one of the classic unsolved problems, which has drawn much interest in the context of cuprate high-temperature superconductors [1] , [2] , [3] . In one picture, the single hole forms a coherent QP propagating in a medium of quantum-fluctuating spins, which strongly renormalizes the dispersion relations and the mutual interactions of the holes at finite doping. This spin–polaron picture is supported by numerical approaches, such as quantum Monte Carlo [4] , exact diagonalization [5] and self-consistent Born approximation (SCBA) [2] . In a contrasting picture, the notion of QP can break down due to various mechanism such as orthogonality catastrophe [6] , spin–charge separation [7] and/or localization effects [8] , reflecting the unconventional nature of two-dimensional (2D), strongly interacting fermions. To date, no evidence for a QP has been found in experiments [9] , [10] , [11] , [12] that probe the dynamics of a single hole doped into a 2D spin–1/2 quantum AFs. Motivated by the recent discovery of a new pseudospin–1/2 Heisenberg AF on a square lattice, Sr 2 IrO 4 (refs 13 , 14 , 15 , 16 , 17 , 18 ), we demonstrate a novel experimental approach using resonant inelastic X-ray scattering (RIXS), which is a rapidly evolving tool especially well suited for such 5 d transition-metal oxides, to address this longstanding problem. On the basis of its remarkable similarity to superconducting cuprates in structural [18] , electronic [13] and magnetic aspects [14] , [15] , [16] , superconductivity has been predicted in Sr 2 IrO 4 (ref. 19 ). Although the electron correlation strength in Sr 2 IrO 4 has been under much debate [20] , [21] , [22] , [23] , [24] , questioning the validity of classifying this compound as a Mott insulator, Sr 2 IrO 4 shares the same phenomenology that the hole spectral function as measured by angle-resolved photoemission spectroscopy (ARPES) lacks a legitimate QP [13] . This similarity suggests a common origin for the absence of a well-defined QP in the ARPES spectra for two distinct but similar classes of materials. As we shall see, however, Sr 2 IrO 4 supports a well-defined QP in another excitation channel, which RIXS is sensitive to and reflects the same dynamics as that of a hole, offering a novel route to studying elementary excitations in correlated oxides. In an earlier RIXS study of Sr 2 IrO 4 , excitations of a hole across the spin–orbit coupling split levels (from the j =1/2 manifold to the j =3/2 manifold) have been identified and it has been shown that their dispersions can be understood in close analogy to the single-hole problem [16] . 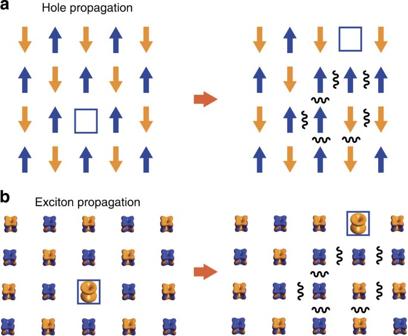Figure 1: Hole versus exciton propagation in an antiferromagnetic background. (a) A moving hole (blue square) leaves a string of excited spins behind; that is, every hopping motion of the hole generates a flipping of a spin relative to the ground state configuration. Black wavy lines indicate pairs of ‘misaligned’ spins. (b) An analogous exciton hopping. While the nature of the spin–orbit exciton (charge-neutral object) and the hole (charged particle) is quite different, they share in common that their hopping creates a string of flipped spins (or isospins in the case of exciton). SeeFig. 2for the description of the isospins and the spin–orbit excitons. Figure 1 depicts the hole-versus-exciton analogy: a ‘foreign’ object injected into a quantum Heisenberg AF, be it a hole or an exciton, creates a string of flipped spins along its hopping path. This analogy, in principle, suggests that the dynamics of a particle moving in a magnetic medium can also be studied using the exciton. However, the energy resolution of RIXS used in the earlier study (≈130 meV) was insufficient to resolve the dispersion and the intrinsic linewidth of the two-exciton modes associated with the two pairs of Kramers doublets in the j =3/2 manifold ( Fig. 2a ). Here we exploit the different orbital symmetries of the two-exciton modes to selectively probe each mode, and with the much improved energy resolution (≈30 meV) offered by RIXS after recent developments, reveal their full dynamics. Figure 1: Hole versus exciton propagation in an antiferromagnetic background. ( a ) A moving hole (blue square) leaves a string of excited spins behind; that is, every hopping motion of the hole generates a flipping of a spin relative to the ground state configuration. Black wavy lines indicate pairs of ‘misaligned’ spins. ( b ) An analogous exciton hopping. While the nature of the spin–orbit exciton (charge-neutral object) and the hole (charged particle) is quite different, they share in common that their hopping creates a string of flipped spins (or isospins in the case of exciton). See Fig. 2 for the description of the isospins and the spin–orbit excitons. 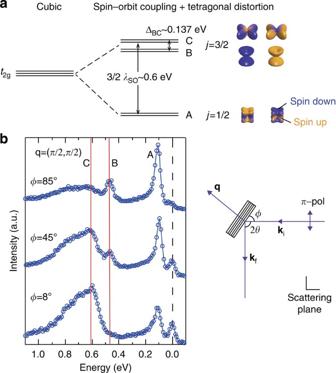Figure 2: RIXS spectra of Sr2IrO4. (a) The spin–orbital level scheme of the three Kramers pairs and their orbital shapes in Sr2IrO4. The three-fold degenerate orbital states oft2gsymmetry under the cubic crystal field splits into aj=1/2 doublet and aj=3/2 quartet in the presence of spin–orbit coupling. The spin–orbit entangled nature of these quantum states is illustrated with colours; orange (blue) represent spin up (down) projection. A tetragonal crystal field further splits thej=3/2 quartet into two Kramers doublets labelled as B and C; B (C) represents states withjzquantum numbers ±3/2 (±1/2). Spin–orbit exciton refers to an excitation of a hole from thej=1/2 manifold to thej=3/2 manifold. (b) Spectrum atq=(π/2,π/2) measured at three different X-ray incident angleϕof 8°, 45° and 82°, corresponding to three-dimensionalqof (−3.5,3,25.5), (0.5,0,34) and (3.5,3,25.5), respectively, in reciprocal lattice units. A, B and C denote the energy positions of the three Kramers pairs illustrated ina. The scattering angle 2θwas kept within 5° from 90°. Full size image Figure 2: RIXS spectra of Sr 2 IrO 4 . ( a ) The spin–orbital level scheme of the three Kramers pairs and their orbital shapes in Sr 2 IrO 4 . The three-fold degenerate orbital states of t 2g symmetry under the cubic crystal field splits into a j =1/2 doublet and a j =3/2 quartet in the presence of spin–orbit coupling. The spin–orbit entangled nature of these quantum states is illustrated with colours; orange (blue) represent spin up (down) projection. A tetragonal crystal field further splits the j =3/2 quartet into two Kramers doublets labelled as B and C; B (C) represents states with j z quantum numbers ±3/2 (±1/2). Spin–orbit exciton refers to an excitation of a hole from the j =1/2 manifold to the j =3/2 manifold. ( b ) Spectrum at q =( π /2, π /2) measured at three different X-ray incident angle ϕ of 8°, 45° and 82°, corresponding to three-dimensional q of (−3.5,3,25.5), (0.5,0,34) and (3.5,3,25.5), respectively, in reciprocal lattice units. A, B and C denote the energy positions of the three Kramers pairs illustrated in a . The scattering angle 2 θ was kept within 5° from 90°. Full size image Strong modulation of RIXS intensities as a function of incident X-ray angle Figure 2b shows the RIXS spectra measured at three different incident angles ϕ of X-ray while fixing momentum transfer at q =( π /2, π /2). The two-exciton modes, labelled as peaks B and C, show strong modulations in intensity as a function of ϕ through the change in the incident and outgoing X-ray polarizations relative to the sample surface and thereby the RIXS matrix elements. In particular, the peak B is strongly enhanced (completely suppressed) by tuning ϕ to normal (grazing) incidence geometry. This strong matrix element effect enables selective mapping of B and C modes, as shown in Fig. 3a . While both B and C modes display rather similar dispersions, the B mode has a much narrower linewidth (see Fig. 4c ). We note that the electron–hole continuum having a threshold of ≈0.41 eV (ref. 25 ) may strongly damp the C mode. With the two-exciton modes disentangled, our high-resolution measurement yields for the B mode a bandwidth of ≈112 meV. This finding is consistent with the expectation that the bandwidth is on the scale of a few times the antiferromagnetic exchange coupling J of about 60 meV (ref. 16 ). The global topology of the dispersions with minimum at q =( π /2, π /2) and maximum at the Γ point precisely matches that measured for a hole in cuprates by ARPES [9] , which strongly supports the hole-versus-exciton analogy. 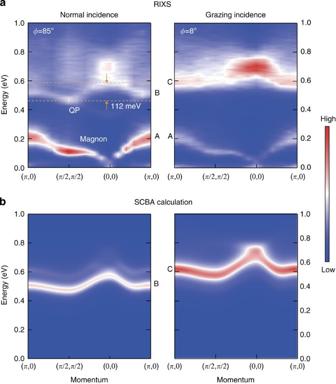Figure 3: Selective mapping of the two-exciton modes and their comparison to SCBA calculations. (a) Image plot of RIXS spectra measured along high-symmetry lines in the normal and grazing incidence geometry. (b) SCBA calculations using the parametersλSO=382 meV, ΔBC=137 meV,t1=J1/2=30 meV,t2=t3=7.6 meV,J1=60 meV,J2=−20 meV andJ3=15 meV.t1,2,3(J1,2,3) denote first, second and third nearest neighbour hoppings (magnetic couplings).λSOand ΔBCare defined inFig. 2. The spectral functions obtained by SCBA calculations are convoluted with a Lorentzian function with 5 meV width. Figure 3: Selective mapping of the two-exciton modes and their comparison to SCBA calculations. ( a ) Image plot of RIXS spectra measured along high-symmetry lines in the normal and grazing incidence geometry. ( b ) SCBA calculations using the parameters λ SO =382 meV, Δ BC =137 meV, t 1 = J 1 /2=30 meV, t 2 = t 3 =7.6 meV, J 1 =60 meV, J 2 =−20 meV and J 3 =15 meV. t 1,2,3 ( J 1,2,3 ) denote first, second and third nearest neighbour hoppings (magnetic couplings). λ SO and Δ BC are defined in Fig. 2 . The spectral functions obtained by SCBA calculations are convoluted with a Lorentzian function with 5 meV width. 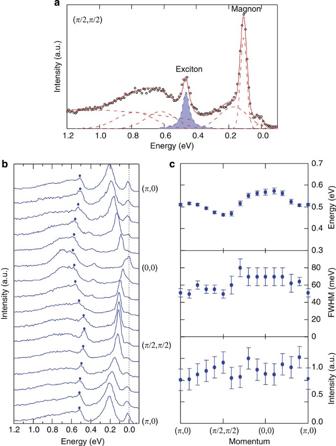Figure 4: Exciton dynamics in Sr2IrO4. (a) RIXS spectrum atq=(π/2,π/2) (black open circles). The blue shaded peak corresponds to the exciton QP peak. The spectrum was fitted (red solid curve) using a Lorenzian lineshape for the exciton QP peak and Gaussian lineshapes for all other peaks (red dashed lines). The low-energy features relative to exciton QP consist of elastic, single- and double-magnon peaks, and high-energy features the sum of C mode and background due to electron–hole continuum and the incoherent part of B mode. (b) Stack plot of the image plot inFig. 2a, left panel. Oval symbols mark the energy position of the QP. In addition to the QP, a small peak with the dispersion minimum at the Γ point atE≈0.37 eV is observed. A similar peak has been observed in a related material Na2IrO3and attributed to a bound state at the edge of the particle–hole continuum29. (c) Energy, width and intensity of the QP peaks along high-symmetry lines extracted from peak fitting as exemplified ina. Error bars represent the s.d. in the data fitting procedure. Full size image Figure 4: Exciton dynamics in Sr 2 IrO 4 . ( a ) RIXS spectrum at q =( π /2, π /2) (black open circles). The blue shaded peak corresponds to the exciton QP peak. The spectrum was fitted (red solid curve) using a Lorenzian lineshape for the exciton QP peak and Gaussian lineshapes for all other peaks (red dashed lines). The low-energy features relative to exciton QP consist of elastic, single- and double-magnon peaks, and high-energy features the sum of C mode and background due to electron–hole continuum and the incoherent part of B mode. ( b ) Stack plot of the image plot in Fig. 2a , left panel. Oval symbols mark the energy position of the QP. In addition to the QP, a small peak with the dispersion minimum at the Γ point at E ≈0.37 eV is observed. A similar peak has been observed in a related material Na 2 IrO 3 and attributed to a bound state at the edge of the particle–hole continuum [29] . ( c ) Energy, width and intensity of the QP peaks along high-symmetry lines extracted from peak fitting as exemplified in a . Error bars represent the s.d. in the data fitting procedure. Full size image Justification of hole-versus-excition analogy We compare the experimental data to the spectral function of the effective t–J model calculated within the SCBA ( Fig. 3b and Supplementary Fig. 1 ). For details, see Supplementary Note 1 and ref. 16 . The calculation yields two modes, one of which is predominantly from the Kramers doublet with quantum numbers | j =3/2, j z =±3/2>, while the other has mostly | j =3/2, j z =±1/2> character. Through an explicit calculation of the RIXS matrix elements, we find that their dependences on ϕ are such that the j z =±1/2 ( j z =±3/2) states, with more in-plane components, are enhanced in intensity in the grazing (normal) incidence geometry. This implies a level scheme of j z =±1/2 lying higher in energy (in the hole picture) than the j z =±3/2 states, which is opposite to expectations based on perfectly cubic or c axis-elongated oxygen octahedra, but agrees with the results from non-resonant inelastic X-ray scattering [26] , electron spin resonance [27] and quantum chemistry calculations [28] . Taking a crystal field splitting Δ BC of 137 meV and fixing all other parameters to values inferred from independent studies, the effective t–J model reproduces the gross features of the experimental spectra. Details are improved by including further neighbouring hoppings, which are expected to be significant based on sizable further neighbour magnetic couplings [16] . With the parameters given in Fig. 3b caption, we find an excellent agreement with the data in terms of the polarization dependence and the dispersion relations, confirming that the exciton dynamics is essentially captured by the effective t–J model. A well-defined excitonic QP in a 2D spin–1/2 quantum AF Having justified the hole-versus-exciton analogy, we now bring to light the key observation from the exciton spectra. The energy distribution curves, measured in the normal incidence geometry to highlight the B mode, reveal a very sharp exciton peak, most prominent at q =( π /2, π /2) ( Fig. 4a ) and resolved throughout most part of the Brillouin zone ( Fig. 4b ). We use a phenomenological Lorentzian lineshape to fit the spectra to extract the peak energy, width and intensity, which are summarized in Fig. 4c . We note that the peak width is as narrow as ≈50 meV (of which 40 meV is intrinsic after deconvoluting the instrumental broadening) at q =( π /2, π /2). While such a sharp peak is not uncommon in RIXS spectra of iridates [29] , it is certainly much narrower than that of the sharpest peak (~200 meV) in the hole spectral function measured by ARPES for the same material [13] , [30] . The peak width is also much smaller than its total bandwidth (≈112 meV), which establishes the exciton as a propagating mode in a solid, or a QP. More importantly, our observation of an excitonic QP establishes hard evidence that a particle can propagate coherently through a 2D spin–1/2 quantum AF. Although dispersive excitons have been observed in classical three-dimensional magnets [31] , [32] , [33] , we are not aware of any excitonic QP observed in a 2D spin–1/2 quantum AF. This raises a fundamental question: why is a QP absent for the single-hole excitation? Thus far we have focused on the similarity between the dynamics of a hole and an exciton. Let us now discuss some important differences. A hole is a charge monopole and its sudden creation in the ARPES process leads to deformation of the surrounding ionic oxygen cage, which results in a strong hole–lattice coupling detrimental for the hole propagation. Further, a hole interacts with charged impurities always present and poorly screened in an insulator. Both of these effects have been shown to strongly damp or wash out sharp QPs [34] , [35] , [36] , thereby significantly redistributing the hole spectral function. In fact, most likely for these reasons, for a quasi-one-dimensional system Sr 2 CuO 3 in which the phenomenon of spin–charge/orbital separation is established [37] , [38] , ARPES measures much-broadened spectra [39] , [40] of the theoretically predicted sharp edge-singularity in the exactly solvable model. By contrast, a charge-neutral exciton with a quadrupole moment should couple much more weakly to the lattice and is not subject to long-range Coulomb forces due to impurities. Thus, the exciton avoids these ‘side effects’ and reveals the intrinsic dynamics of the t–J model that have remained elusive for the past several decades. Our central message is that the unprecedentedly narrow linewidth of the QP allows a direct access into the nature of a QP living in the background of a 2D quantum spin–1/2 Heisenberg AF, and thus that it allows direct verification of a class of theories that predict a finite QP residue in the Mott insulating phase, which has thus far remained inconclusive in the apparent absence of a QP in the hole channel. For instance, the observed exciton intensity can be compared with that calculated in theoretical models on a quantitative level. 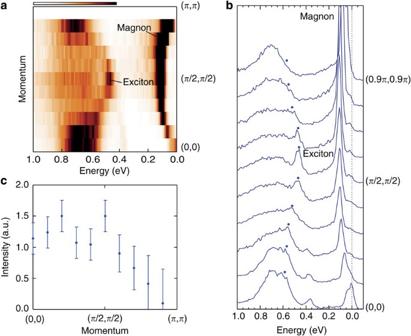Figure 5: Asymmetric exciton QP intensity. (a) Image plot of RIXS spectra along (0,0)–(π,π) direction. (b) Stack plot of the image plot ina. Oval symbols mark the energy position of the QP. (c) Intensity of the QP peaks along (0,0)–(π,π) direction. Error bars represent the s.d. in the data fitting procedure. Figure 5a,b shows the exciton dispersion along (0,0)–( π , π ) direction. The dispersion is symmetric with respect to ( π /2, π /2) point on the magnetic zone boundary, but the intensities inside and outside of the magnetic zone differ significantly ( Fig. 5c ); the exciton QP displays a steep drop in intensity as ( π /2, π /2) is crossed. This is a generic feature predicted for a hole in a t – J model within an SCBA approach [41] and indirectly inferred from ARPES measurements on cuprates [42] . Although some deviations from the cuprate physics might have been expected on general grounds due to fundamentally different nature of a hole and an exciton, and material-specific differences between Sr 2 IrO 4 and cuprates, the striking agreement down to a level of fine details with theories constructed for hole dynamics in cuprates demonstrates excellent parallel between the low-energy physics of Sr 2 IrO 4 and the cuprates. Figure 5: Asymmetric exciton QP intensity. ( a ) Image plot of RIXS spectra along (0,0)–( π , π ) direction. ( b ) Stack plot of the image plot in a . Oval symbols mark the energy position of the QP. ( c ) Intensity of the QP peaks along (0,0)–(π, π ) direction. Error bars represent the s.d. in the data fitting procedure. Full size image RIXS measurements A single crystal of Sr 2 IrO 4 of 1 mm × 1 mm size grown by the flux method was mounted in a displex closed-cycle cryostat and measured at 15 K. The RIXS measurements were performed using the MERIX spectrometer at the 30-ID beamline [43] of the Advanced Photon Source. X-rays were monochromatized to a bandwidth of 15 meV, and focused to have a beam size of 45(H) × 30(V) μm 2 . A horizontal scattering geometry was used with the incident photon polarization in the scattering plane. A Si (844) diced spherical analyser with 4 inch radius and a position-sensitive silicon microstrip detector were used in the Rowland geometry. The overall energy resolution of the MERIX spectrometer at the Ir L 3 edge was 30 meV, as determined from the full-width-half-maximum of the elastic peak. The RIXS spectra were reproduced at least twice to check for consistency. How to cite this article: Kim, J. et al. Excitonic quasiparticles in a spin–orbit Mott insulator. Nat. Commun. 5:4453 doi: 10.1038/ncomms5453 (2014).